Divergent mutational processes distinguish hypoxic and normoxic tumours Many primary tumours have low levels of molecular oxygen (hypoxia), and hypoxic tumours respond poorly to therapy. Pan-cancer molecular hallmarks of tumour hypoxia remain poorly understood, with limited comprehension of its associations with specific mutational processes, non-coding driver genes and evolutionary features. Here, as part of the ICGC/TCGA Pan-Cancer Analysis of Whole Genomes (PCAWG) Consortium, which aggregated whole genome sequencing data from 2658 cancers across 38 tumour types, we quantify hypoxia in 1188 tumours spanning 27 cancer types. Elevated hypoxia associates with increased mutational load across cancer types, irrespective of underlying mutational class. The proportion of mutations attributed to several mutational signatures of unknown aetiology directly associates with the level of hypoxia, suggesting underlying mutational processes for these signatures. At the gene level, driver mutations in TP53 , MYC and PTEN are enriched in hypoxic tumours, and mutations in PTEN interact with hypoxia to direct tumour evolutionary trajectories. Overall, hypoxia plays a critical role in shaping the genomic and evolutionary landscapes of cancer. Approximately half of all solid tumours are characterized by low levels of molecular oxygen (hypoxia) [1] , [2] , [3] , [4] . Sub-regions of hypoxia can result from disrupted oxygen supply: irregular and disorganized tumour vasculature can reduce oxygen availability [5] . Hypoxia can also be caused by changes in oxygen demand: altered tumour metabolism [6] , [7] can increase intra-cellular demand for oxygen, potentially extending hypoxia signalling to liquid tumours. The adaptation of tumour cells to this imbalance in oxygen supply and demand is associated with poor clinical prognosis in several cancer types, attributed at least in part to hypoxia-associated genomic instability and clonal selection [8] , [9] , [10] , [11] , [12] , [13] , [14] , [15] , [16] . Previous work has provided insight into the molecular origins and consequences of tumour hypoxia and genomic instability. Dynamic cycling of hypoxia can select for cells with TP53 mutations and for those that are apoptosis-deficient [17] , [18] . Indeed mutations in TP53 occur at a higher frequency in hypoxic primary tumours of at least 9 types [16] . The abundance of proteins involved in homologous recombination (e.g. RAD51) and non-homologous end joining (e.g. Ku70) are reduced under hypoxia, and these changes can persist for 2 days after reoxygenation [19] , [20] , [21] . Genes central to efficient mismatch repair (e.g. MLH1 and MSH2 ) are also downregulated under hypoxia [22] , [23] . Further, co-presence of tumour hypoxia and high genomic instability [14] , [15] , specific cellular morphologies like intraductal and cribriform carcinoma [24] or specific mutations like loss of PTEN [16] , synergistically predict for rapid relapse after definitive local therapy in some tumour types, particularly prostate cancer. These data underscore the relationship between hypoxia and DNA repair defects, and suggest the tumour microenvironment applies a selective pressure leading to the development of specific genomic profiles. We previously evaluated the exomic and copy-number alteration (CNA) consequences of tumour hypoxia across 19 cancer types [16] . However, the influence of tumour hypoxia on pan-cancer driver alterations, mutational signatures, and subclonal architectures remains unclear. To fill this gap, we calculated tumour hypoxia scores for 1188 tumours with whole-genome sequencing (WGS) and RNA sequencing, spanning 27 cancer types. Genome sequencing data was aggregated by the Pan-Cancer Analysis of Whole Genomes (PCAWG) consortium and generated by the ICGC and TCGA projects. These sequencing data were re-analyzed with standardized, high-accuracy pipelines to align to the human genome (reference build hs37d5) and identify germline variants and somatic mutations, as described previously [25] . This sequencing data together with our high-quality hypoxia quantitation represents a powerful hypothesis-generating mechanism to suggest useful back-translational in vitro experiments and better define the hypoxia-associated mutator phenotype across cancers. We associated hypoxia with key driver alterations in coding and non-coding regions of the genome, and find hypoxia is associated with specific mutational signatures of unknown aetiology. We illustrate the joint impact of PTEN and the tumour microenvironment in influencing the evolutionary trajectory of tumours. Overall, these data highlight the genomic changes through which hypoxia drives aggressive cancers. The pan-cancer landscape of tumour hypoxia We compiled a cohort of 1188 tumours from 27 cancer types via the PCAWG Consortium. All samples had matched tumour and reference normal WGS and tumour RNA sequencing data generated by the ICGC and TCGA projects. WGS [25] and RNA-sequencing [26] analyses were systematically carried out by centralized teams with consistent and high-accuracy bioinformatics pipelines. Normal reference samples had a mean WGS coverage of 39 reads per base-pair while coverage for tumour samples had a bimodal distribution with modes at 38 and 60 reads per base-pair [25] . All samples underwent an extensive and systematic quality assurance process [25] . We used linear mixed-effect models to associate hypoxia with features of interest across cancers while adjusting for tumour purity, age, and sex [27] , [28] . Cancer type was further incorporated as a random effect in every model, allowing us to consider a different baseline value for the feature of interest for each cancer type. As a measure of effect size we report conditional R 2 values, denoted as \(R_{{{\mathrm{{{LMEM - C}}}}}}^2\) , which reflect the variance explained by the fixed and random factors in each model [29] . We also report marginal R 2 values, denoted as \(R_{{{\mathrm{{{LMEM - M}}}}}}^2\) , which reflect the variance explained only by the fixed factors [29] . We scored tumour hypoxia in all 1188 tumours using a trio of mRNA-based hypoxia signatures from Buffa [30] , Winter [31] and Ragnum [32] (Fig. 1a , Supplementary Fig. 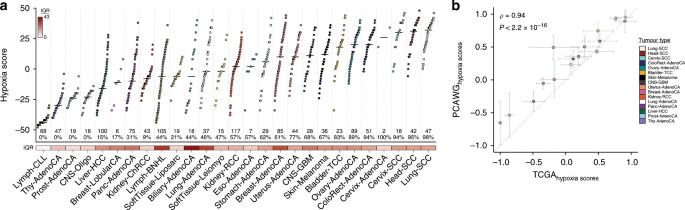Fig. 1: The pan-cancer landscape of tumour hypoxia. We quantified tumour hypoxia in 1188 independent tumours spanning 27 different cancer types.aHypoxia scores for 27 types of cancer, based on the Buffa mRNA abundance signature. Cancer types are sorted by the median hypoxia score (horizontal black line) for each cancer type. Each dot represents one tumour. Sample sizes for each cancer type are listed near the bottom along with the percent of tumours that have elevated hypoxia (hypoxia score > 0). The variability in hypoxia within cancer types was measured by the interquartile range (IQR), shown along the bottom. The IQR was particularly high in biliary adenocarcinoma (IQR = 43.0; Biliary-AdenoCA), lymphoid B-cell non-Hodgkin’s lymphomas (IQR = 36.0; Lymph-BNHL), lung adenocarcinoma (IQR = 34.0; Lung-AdenoCA) and breast adenocarcinoma (IQR = 32; Breast-AdenoCA). By contrast, chronic lymphocytic leukaemia (IQR = 2.0; Lymph-CLL) and thyroid adenocarcinoma (IQR = 11.0; Thy-AdenoCA) showed less variance in hypoxia score.bAnalysis of hypoxia between 16 comparable cancer types in PCAWG and TCGA (Spearman’sρ, AS89). Dots represent the mean of the scaled median hypoxia scores from three different mRNA-based hypoxia signatures. Error bars represent the standard deviation of the scaled median hypoxia scores. Overall, the pan-cancer quantification of hypoxia between the PCAWG and TCGA datasets shows strong agreement. 1a, b , Supplementary Table 1 , Supplementary Data 1 ). Hypoxia scores from each of these independent signatures were strongly correlated ( ρ = 0.71–0.88, all p < 2.2 × 10 −16 , AS89; Supplementary Fig. 1c ) and consistently predicted squamous tumours of the lung (Lung-SCC), cervix (Cervix-SCC), and head (Head-SCC) as the most hypoxic (Supplementary Fig. 1d, e ). Comparatively, chronic lymphocytic leukaemias (Lymph-CLL) and thyroid adenocarcinomas (Thy-AdenoCA) were the least hypoxic, consistent with previous [16] reports ( ρ = 0.94, p < 2.2 × 10 −16 , AS89; Fig. 1b , Supplementary Fig. 1f, h ). Remarkably, subsets of patients from 23/27 cancer types have tumours with elevated hypoxia (hypoxia score > 0) and tumours consistently have elevated hypoxia compared to normal tissues (Supplementary Fig. 2a–c ). Fig. 1: The pan-cancer landscape of tumour hypoxia. We quantified tumour hypoxia in 1188 independent tumours spanning 27 different cancer types. a Hypoxia scores for 27 types of cancer, based on the Buffa mRNA abundance signature. Cancer types are sorted by the median hypoxia score (horizontal black line) for each cancer type. Each dot represents one tumour. Sample sizes for each cancer type are listed near the bottom along with the percent of tumours that have elevated hypoxia (hypoxia score > 0). The variability in hypoxia within cancer types was measured by the interquartile range (IQR), shown along the bottom. The IQR was particularly high in biliary adenocarcinoma (IQR = 43.0; Biliary-AdenoCA), lymphoid B-cell non-Hodgkin’s lymphomas (IQR = 36.0; Lymph-BNHL), lung adenocarcinoma (IQR = 34.0; Lung-AdenoCA) and breast adenocarcinoma (IQR = 32; Breast-AdenoCA). By contrast, chronic lymphocytic leukaemia (IQR = 2.0; Lymph-CLL) and thyroid adenocarcinoma (IQR = 11.0; Thy-AdenoCA) showed less variance in hypoxia score. b Analysis of hypoxia between 16 comparable cancer types in PCAWG and TCGA (Spearman’s ρ , AS89). Dots represent the mean of the scaled median hypoxia scores from three different mRNA-based hypoxia signatures. Error bars represent the standard deviation of the scaled median hypoxia scores. Overall, the pan-cancer quantification of hypoxia between the PCAWG and TCGA datasets shows strong agreement. Full size image Considering the strong agreement between the Winter, Buffa and Ragnum hypoxia signatures (Fig. 1a , Supplementary Fig. 1c, d ), we used the Buffa signature for subsequent analyses. The Buffa signature has been previously used for pan-cancer analyses and shows results consistent with those from other signatures [16] . We first assessed the degree of inter-tumoural heterogeneity in hypoxia that lies within individual cancer types rather than between them. Over 42% of the variance in hypoxia scores occurs within individual cancer types, highlighting the microenvironmental diversity between tumours arising in a single tissue. This variability in hypoxia score within cancer types was especially elevated in some tumour types, particularly biliary adenocarcinomas (interquartile range, IQR = 43.0; Biliary-AdenoCA), mature B-cell lymphomas (IQR = 36.0; Lymph-BNHL), lung adenocarcinomas (IQR = 34.0; Lung-AdenoCA) and breast adenocarcinomas (IQR = 32.0; Breast-AdenoCA). This was in contrast to chronic lymphocytic leukaemias (IQR = 2.0; Lymph-CLL) and prostate adenocarcinomas (IQR = 6.0; Prost-AdenoCA) where little inter-tumoural variability in hypoxia was observed. The variability in hypoxia score was not significantly associated with the median hypoxia score within cancer types ( ρ = 0.20, p = 0.30, AS89; Supplementary Fig. 2d ) or with sample size ( ρ = 0.22, p = 0.27, AS89; Supplementary Fig. 2e ). Overall, extensive heterogeneity exists in hypoxia levels within and across cancer types. The genomic correlates of tumour hypoxia To determine whether genomic instability arising from specific mutational classes is associated with hypoxia, we looked to identify hypoxia-associated pan-cancer mutational density and summary features [33] . As a positive control, we first considered the p ercentage of the g enome with a copy-number a berration (PGA), an engineered feature that is a surrogate for genomic instability and is associated with hypoxia across several tumour types [16] (Supplementary Fig. 2f ). Indeed, in this diverse pan-cancer cohort, hypoxic tumours have elevated genomic instability while controlling for cancer type, tumour purity, age and sex [27] ( p = 2.41 × 10 −8 , \(R_{{{\mathrm{{{LMEM - M}}}}}}^2\) = 0.022, \(R_{{{\mathrm{{{LMEM - C}}}}}}^2\) = 0.57, linear mixed-effect model; Fig. 2a ). Fig. 2: The genomic correlates of tumour hypoxia. We associated tumour hypoxia with mutational density and summary features, a , and driver mutations, b , across 27 cancer types using linear mixed-effect models. Hypoxia scores for all 1188 tumours are shown along the top. a Elevated tumour hypoxia was strongly associated with more deletions, elevated PGA, smaller CNAs, and a higher number of SNVs per megabase ( n = 1188 independent tumours). Bonferroni-adjusted p -values are shown on the right. b We tested if driver mutations (e.g. any of SNV, CNA, SV or a compound event with more than one type of mutation) were associated with hypoxia in 1096 independent tumours with driver mutation data. Tumours with mutations in BCL2 showed lower levels of hypoxia while patients with mutations in TP53 showed remarkably elevated tumour hypoxia. Other driver mutations associated with elevated hypoxia include the oncogene MYC and the tumour suppressor PTEN . FDR-adjusted p -values are shown along the right. SV structural variant; PGA percentage of the genome with a copy-number aberration; CNA copy-number aberration; SNV single nucleotide variant; H-H head-to-head; T-T tail-to-tail. All associations were modelled using linear mixed-effect models while adjusting for cancer type, tumour purity, age and sex. Full size image We then considered the association of hypoxia scores with 14 other metrics of the mutation density of CNAs, structural variants (SVs) and single nucleotide variants (SNVs) using linear mixed-effect models (Fig. 2a , Supplementary Fig. 2f , Supplementary Tables 2 , 3 ). The strongest single correlate of tumour hypoxia was the total number of deletions, where patients with elevated hypoxia had more deletions ( p = 1.11 × 10 −10 , \(R_{{{\mathrm{{{LMEM - M}}}}}}^2\) = 0.023, \(R_{{{\mathrm{{{LMEM - C}}}}}}^2\) = 0.59, linear mixed-effect model). Elevated numbers of other SVs such as duplications ( p = 2.94 × 10 −4 , \(R_{{{\mathrm{{{LMEM - M}}}}}}^2\) = 0.0084, \(R_{{{\mathrm{{{LMEM - C}}}}}}^2\) = 0.60, linear mixed-effect model) and truncations ( p = 3.29 × 10 −3 , \(R_{{{\mathrm{{{LMEM - M}}}}}}^2\) = 0.0062, \(R_{{{\mathrm{{{LMEM - C}}}}}}^2\) = 0.60, linear mixed-effect model) were also associated with high hypoxia, and we confirmed this within individual cancer types (Supplementary Fig. 3a ). Other features associated with elevated hypoxia include smaller CNAs ( p = 3.51 × 10 −3 , \(R_{{{\mathrm{{{LMEM - M}}}}}}^2\) = 0.0065, \(R_{{{\mathrm{{{LMEM - C}}}}}}^2\) = 0.59, linear mixed-effect model) and more SNVs/Mbp ( p = 5.55 × 10 −3 , \(R_{{{\mathrm{{{LMEM - M}}}}}}^2\) = 0.0054, \(R_{{{\mathrm{{{LMEM - C}}}}}}^2\) = 0.60, linear mixed-effect model). Since mutational density features can be correlated, we wanted to further test if SNVs per megabase were independently associated with hypoxia after adjusting for the total number of deletions. We created a linear mixed-effect model associating hypoxia with the number of SNVs per megabase while adjusting for cancer type, age, sex, tumour purity and the number of deletions. We also created a second model which lacked our feature of interest, SNVs per megabase, and compared the two models using an ANOVA (see the “Methods” section). The p -value for this comparison was 0.011, suggesting that the number of SNVs per megabase are associated with hypoxia independent of the number of deletions (and other potential confounders included in the models). Overall, hypoxia is associated with increased numbers of most types of somatic mutations. 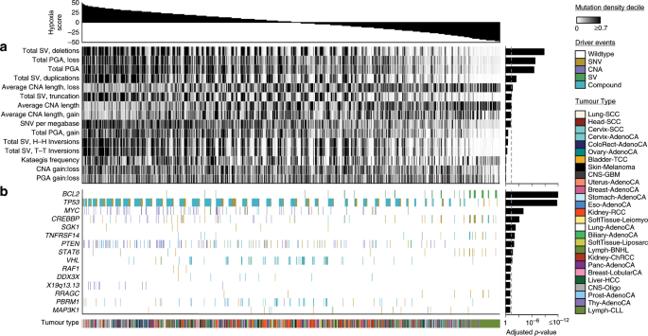Fig. 2: The genomic correlates of tumour hypoxia. We associated tumour hypoxia with mutational density and summary features,a, and driver mutations,b, across 27 cancer types using linear mixed-effect models. Hypoxia scores for all 1188 tumours are shown along the top.aElevated tumour hypoxia was strongly associated with more deletions, elevated PGA, smaller CNAs, and a higher number of SNVs per megabase (n= 1188 independent tumours). Bonferroni-adjustedp-values are shown on the right.bWe tested if driver mutations (e.g. any of SNV, CNA, SV or a compound event with more than one type of mutation) were associated with hypoxia in 1096 independent tumours with driver mutation data. Tumours with mutations inBCL2showed lower levels of hypoxia while patients with mutations inTP53showed remarkably elevated tumour hypoxia. Other driver mutations associated with elevated hypoxia include the oncogeneMYCand the tumour suppressorPTEN. FDR-adjustedp-values are shown along the right. SV structural variant; PGA percentage of the genome with a copy-number aberration; CNA copy-number aberration; SNV single nucleotide variant; H-H head-to-head; T-T tail-to-tail. All associations were modelled using linear mixed-effect models while adjusting for cancer type, tumour purity, age and sex. Considering the strong association of hypoxia with mutational density, we next looked to determine if these were only general effects or selectively affected specific genes or chromosome regions. We leveraged a catalogue of 653 driver mutations [25] , with CNA, SV and SNV data available for 1096 patients. In cases where a patient had multiple mutations in the same gene (e.g. a CNA and an SNV) we denoted these as compound events. We again used linear-mixed effect models to associate hypoxia with each driver feature across cancers (Fig. 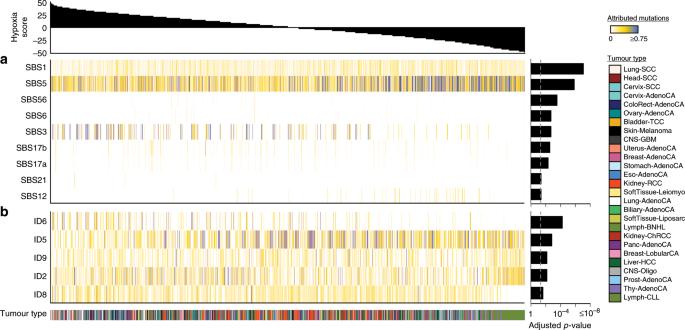Fig. 3: Hypoxia-associated mutational signatures. We associated hypoxia with the proportion of mutations attributed to specific mutational signatures using linear-mixed effect models. Hypoxia scores for 1188 independent tumours are shown across the top while FDR-adjustedp-values are shown on the right.aHypoxia was associated with a series of single base substitution signatures with unknown aetiology including SBS5, SBS17a, SBS17b and SBS12. Some of these mutational signatures may reflect hypoxia-dependent mutational processes. Hypoxia was also associated with a lower proportion of attributed mutations to SBS1, which reflects deamination of 5-methylcytosine, and a higher proportion of attributed mutations to SBS3, which is related to deficiencies in DNA double-strand break repair and homologous recombination.bSeveral signatures of small insertions and deletions were also associated with hypoxia, including ID6 and ID2, which reflect defective homologous recombination and defective DNA mismatch repair, respectively. ID5, ID9 and ID4, all with unknown aetiology, were significantly associated with hypoxia score. All associations were modelled using linear-mixed effect models while adjusting for cancer type, tumour purity, age and sex. 2b ). Adjusting for cancer type, tumour purity, age and sex, 10 driver events were associated with hypoxia across cancers (FDR < 0.10, linear-mixed effect models; Supplementary Fig. 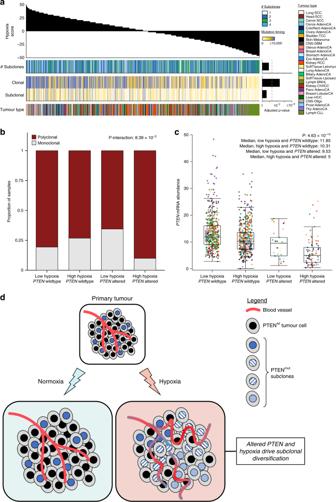Fig. 4: The subclonal hallmarks of tumour hypoxia. We associated tumour hypoxia with features related to the subclonal architecture of 1188 independent tumours from 27 cancer types using linear mixed-effect models.aHypoxia scores are shown along the top while Bonferroni-adjustedp-values are shown on the right. Hypoxia was not associated with the number of subclones in the tumour but elevated hypoxia was associated with a higher number of clonal mutations.bWe also observed a significant interaction between hypoxia and alteredPTENwhere tumours with both of these features were particularly likely to be polyclonal.cThe mRNA abundance ofPTENis modulated by bothPTENmutational status and tumour hypoxia. Tumours with alteredPTENand elevated hypoxia have the lowest abundance ofPTENmRNA. mRNA abundance is reported as FPKM with upper-quartile normalization. A Tukey box plot is shown. Box plots represent the median (centre line) and upper and lower quartiles (box limits), and whiskers extend to the minimum and maximum values within 1.5× the interquartile range. All associations were modelled using linear mixed-effect models while adjusting for cancer type, tumour purity, age and sex.dAlteredPTENand hypoxia may drive subclonal diversification. Many primary tumours have elevated hypoxia due to increased demand or decreased supply of oxygen. Tumours with elevated hypoxia tend to have alteredPTEN. Elevated hypoxia and alteredPTENmay drive subclonal diversification and poor outcomes. 2f , Supplementary Table 4 ). Tumours with mutations in BCL2 (FDR = 7.56 × 10 −15 , \(R_{{{\mathrm{{{LMEM - M}}}}}}^2\) = 0.045, \(R_{{{\mathrm{{{LMEM - C}}}}}}^2\) = 0.62, linear-mixed effect model) showed lower levels of hypoxia compared to those without. All alterations of BCL2 in this cohort were SVs, so it is important to note that this association could not be identified from previous exome-sequencing data. Similarly, mutations in the tumour suppressor TP53 were associated with elevated hypoxia across cancers (FDR = 1.97 × 10 −12 , \(R_{{{\mathrm{{{LMEM - M}}}}}}^2\) = 0.043, \(R_{{{\mathrm{{{LMEM - C}}}}}}^2\) = 0.59, linear-mixed effect model), consistent with previous descriptions of hypoxia-mediated selection of TP53 -mutated cells [17] and elevated hypoxia in breast cancers with TP53 mutations [16] . We also confirmed this association within individual cancer types (Supplementary Fig. 3b ). Mutations of the oncogene MYC (FDR = 1.07 × 10 −4 , \(R_{{{\mathrm{{{LMEM - M}}}}}}^2\) = 0.016, \(R_{{{\mathrm{{{LMEM - C}}}}}}^2\) = 0.60, linear-mixed effect model) and tumour suppressor PTEN (FDR = 1.50 × 10 −2 , \(R_{{{\mathrm{{{LMEM - M}}}}}}^2\) = 0.0098, \(R_{{{\mathrm{{{LMEM - C}}}}}}^2\) = 0.59, linear mixed-effect model) were also associated with elevated hypoxia. Alterations in mitochondrial genes [34] were not significantly associated with tumour hypoxia (Supplementary Fig. 3c ). Thus, hypoxia is associated with both broad elevation of mutation density of most types of somatic variation, along with a consistent signature of alterations in oncogenes and tumour suppressors across cancers. Hypoxia-associated mutational signatures Previous work has used nonnegative matrix factorization to identify distinct mutational processes in cancer cells from endogenous and exogenous agents [35] . To identify hypoxia-associated mutational processes, we tested if hypoxia score was associated with the proportion of mutations attributed to each mutational signature using linear-mixed effect models. Of the 65 single base substitution (SBS) signatures tested, nine showed differential activity in hypoxic tumours compared to non-hypoxic ones, while controlling for cancer type, tumour purity, age and sex (FDR < 0.10, linear mixed-effect models; Fig. 3a , Supplementary Table 5 ). Of these, six were more active and three less active in tumours with elevated hypoxia. Since previous work has shown that DNA repair is impaired under hypoxia, it was not surprising to observe that a higher proportion of mutations were attributed to SBS3 (related to defective homologous recombination-based repair) in tumours with elevated hypoxia score (FDR = 1.98 × 10 −3 , \(R_{{{\mathrm{{{LMEM - M}}}}}}^2\) = 0.016, \(R_{{{\mathrm{{{LMEM - C}}}}}}^2\) = 0.60, linear-mixed effect model). Further, SBS6 (FDR = 1.98 × 10 −3 , \(R_{{{\mathrm{{{LMEM - M}}}}}}^2\) = 0.0086, \(R_{{{\mathrm{{{LMEM - C}}}}}}^2\) = 0.61, linear-mixed effect model) and SBS21 (FDR = 4.31 × 10 −2 , \(R_{{{\mathrm{{{LMEM - M}}}}}}^2\) = 0.0051, \(R_{{{\mathrm{{{LMEM - C}}}}}}^2\) = 0.61, linear-mixed effect model), both related to defective DNA mismatch repair, had a higher proportion of attributed mutations with increasing hypoxia. A lower proportion of mutations were also attributed to SBS1, previously related to the deamination of 5-methylcytosine, with increasing hypoxia (FDR = 8.33 × 10 −8 , \(R_{{{\mathrm{{{LMEM - M}}}}}}^2\) = 0.033, \(R_{{{\mathrm{{{LMEM - C}}}}}}^2\) = 0.61, linear-mixed effect model). Fig. 3: Hypoxia-associated mutational signatures. We associated hypoxia with the proportion of mutations attributed to specific mutational signatures using linear-mixed effect models. Hypoxia scores for 1188 independent tumours are shown across the top while FDR-adjusted p -values are shown on the right. a Hypoxia was associated with a series of single base substitution signatures with unknown aetiology including SBS5, SBS17a, SBS17b and SBS12. Some of these mutational signatures may reflect hypoxia-dependent mutational processes. Hypoxia was also associated with a lower proportion of attributed mutations to SBS1, which reflects deamination of 5-methylcytosine, and a higher proportion of attributed mutations to SBS3, which is related to deficiencies in DNA double-strand break repair and homologous recombination. b Several signatures of small insertions and deletions were also associated with hypoxia, including ID6 and ID2, which reflect defective homologous recombination and defective DNA mismatch repair, respectively. ID5, ID9 and ID4, all with unknown aetiology, were significantly associated with hypoxia score. All associations were modelled using linear-mixed effect models while adjusting for cancer type, tumour purity, age and sex. Full size image Intriguingly, hypoxia was also associated with a number of SBS signatures with unknown aetiology (Fig. 3b ). The strongest of these was SBS5, where elevated hypoxia was associated with a significantly lower proportion of mutations attributed to the signature (FDR = 1.43 × 10 −6 , \(R_{{{\mathrm{{{LMEM - M}}}}}}^2\) = 0.022, \(R_{{{\mathrm{{{LMEM - C}}}}}}^2\) = 0.59, linear-mixed effect model). A significantly lower proportion of mutations were also attributed to SBS12 with increasing hypoxia score (FDR = 4.31 × 10 −2 , \(R_{{{\mathrm{{{LMEM - M}}}}}}^2\) = 0.0066, \(R_{{{\mathrm{{{LMEM - C}}}}}}^2\) = 0.60, linear-mixed effect model). In contrast, a higher proportion of mutations were attributed to SBS17a (FDR = 4.80 × 10 −3 , \(R_{{{\mathrm{{{LMEM - M}}}}}}^2\) = 0.0072, \(R_{{{\mathrm{{{LMEM - C}}}}}}^2\) = 0.61, linear mixed-effect model) and SBS17b (FDR = 2.83 × 10 −3 , \(R_{{{\mathrm{{{LMEM - M}}}}}}^2\) = 0.079, \(R_{{{\mathrm{{{LMEM - C}}}}}}^2\) = 0.61, linear mixed-effect model) with increasing hypoxia. Analysis of small insertion and deletion (ID) signatures illustrated a similar story. Of the 17 ID signatures analyzed, the activity of 5 were associated with tumour hypoxia scores while controlling for cancer type, tumour purity, age and sex (FDR < 0.10, linear mixed-effect models; Fig. 3b , Supplementary Table 6 ). Of these, 3 were more active in tumours with elevated hypoxia while 2 were less active in them. The defective homologous recombination signature ID6 (FDR = 5.76 × 10 −5 , \(R_{{{\mathrm{{{LMEM - M}}}}}}^2\) = 0.015, \(R_{{{\mathrm{{{LMEM - C}}}}}}^2\) = 0.60, linear mixed-effect model) and defective DNA mismatch repair signature ID2 (FDR = 7.06 × 10 −3 , \(R_{{{\mathrm{{{LMEM - M}}}}}}^2\) = 0.011, \(R_{{{\mathrm{{{LMEM - C}}}}}}^2\) = 0.61, linear mixed-effect model) had a higher proportion of attributed mutations as hypoxia score increased. Several signatures with unknown aetiology were also significantly associated with hypoxia score, including ID5 (FDR = 1.54 × 10 −3 , \(R_{{{\mathrm{{{LMEM - M}}}}}}^2\) = 0.016, \(R_{{{\mathrm{{{LMEM - C}}}}}}^2\) = 0.60, linear mixed-effect model) and ID9 (FDR = 7.06 × 10 −3 , \(R_{{{\mathrm{{{LMEM - M}}}}}}^2\) = 0.0068, \(R_{{{\mathrm{{{LMEM - C}}}}}}^2\) = 0.60, linear mixed-effect model). These data suggest that oxygen levels play a direct or indirect role in the accumulation of specific mutations in cancer cells that are reflected by these signatures. The subclonal hallmarks of tumour hypoxia State-of-the-art methods for subclonal reconstruction rely on WGS data [36] , making the PCAWG dataset ideal for understanding the evolutionary pressures imposed by hypoxia. We and others have shown that some mutations consistently occur early during tumourigenesis while others occur later and that hypoxia is associated with CNAs occurring early in localized prostate cancer [16] , [37] , [38] . To explore if this interaction between the tumour microenvironment and mutational landscape exists more broadly in cancer, we assessed if hypoxia was related to the number of clonal or subclonal mutations across 1188 tumours from 27 cancer types [38] . Clonal mutations are common to all cells in a tumour while subclonal ones are only present in a subpopulation of cells. We found that elevated hypoxia was significantly associated with an increased number of clonal alterations across cancers (Bonferroni-adjusted p = 4.65 × 10 −3 , \(R_{{{\mathrm{{{LMEM - M}}}}}}^2\) = 0.0074, \(R_{{{\mathrm{{{LMEM - C}}}}}}^2\) = 0.60, linear mixed-effect model; Fig. 4a , Supplementary Table 7 ), particularly clonal SVs ( p = 1.17 × 10 −5 , \(R_{{{\mathrm{{{LMEM - M}}}}}}^2\) = 0.013, \(R_{{{\mathrm{{{LMEM - C}}}}}}^2\) = 0.60, linear mixed-effect model). In contrast, tumour hypoxia was not significantly associated with the number of subclonal alterations (Bonferroni-adjusted p = 0.28, \(R_{{{\mathrm{{{LMEM - M}}}}}}^2\) = 0.0039, \(R_{{{\mathrm{{{LMEM - C}}}}}}^2\) = 0.60, linear mixed-effect model; Fig. 4a ). Further, consistent with findings in prostate cancer [16] , hypoxia was not associated with the number of subclones detected (Bonferroni-adjusted p = 0.14, \(R_{{{\mathrm{{{LMEM - M}}}}}}^2\) = 0.0051, \(R_{{{\mathrm{{{LMEM - C}}}}}}^2\) = 0.60, linear mixed-effect model; Fig. 4a ). These data suggest that hypoxia applies a selective pressure on tumours during their early evolution, prior to subclonal diversification. Fig. 4: The subclonal hallmarks of tumour hypoxia. We associated tumour hypoxia with features related to the subclonal architecture of 1188 independent tumours from 27 cancer types using linear mixed-effect models. a Hypoxia scores are shown along the top while Bonferroni-adjusted p -values are shown on the right. Hypoxia was not associated with the number of subclones in the tumour but elevated hypoxia was associated with a higher number of clonal mutations. b We also observed a significant interaction between hypoxia and altered PTEN where tumours with both of these features were particularly likely to be polyclonal. c The mRNA abundance of PTEN is modulated by both PTEN mutational status and tumour hypoxia. Tumours with altered PTEN and elevated hypoxia have the lowest abundance of PTEN mRNA. mRNA abundance is reported as FPKM with upper-quartile normalization. A Tukey box plot is shown. Box plots represent the median (centre line) and upper and lower quartiles (box limits), and whiskers extend to the minimum and maximum values within 1.5× the interquartile range. All associations were modelled using linear mixed-effect models while adjusting for cancer type, tumour purity, age and sex. d Altered PTEN and hypoxia may drive subclonal diversification. Many primary tumours have elevated hypoxia due to increased demand or decreased supply of oxygen. Tumours with elevated hypoxia tend to have altered PTEN . Elevated hypoxia and altered PTEN may drive subclonal diversification and poor outcomes. Full size image Next, we assessed if the mutational background of a tumour together with its oxygenation level was linked to its evolutionary trajectory. We previously demonstrated that patients with hypoxic polyclonal prostate tumours with loss of the tumour suppressor PTEN tend to have a poor prognosis [16] . Indeed, here we observed a significant interaction between tumour hypoxia and loss of PTEN in predicting subclonal architecture ( p interaction = 8.39 × 10 −3 , \(R_{{{\mathrm{{{LMEM - M}}}}}}^2\) = 0.60, \(R_{{{\mathrm{{{LMEM - C}}}}}}^2\) = 0.87, linear mixed-effect model; Fig. 4b ). Specifically, tumours with both of these features tend to have a polyclonal architecture across cancers. The downstream impact of this interaction between the genome and the tumour microenvironment was observed in RNA data: tumours with both altered PTEN and elevated hypoxia had the lowest abundance of PTEN mRNA ( p = 4.63 × 10 −14 , \(R_{{{\mathrm{{{LMEM - M}}}}}}^2\) = 0.054, \(R_{{{\mathrm{{{LMEM - C}}}}}}^2\) = 0.47, linear mixed-effect model; Fig. 4c ). Thus, the evolutionary trajectory of a tumour may be driven by the presence of a mutation in a specific microenvironmental context (Fig. 4d ). Hypoxia is a feature of many solid and liquid tumours and is associated with aggressive disease. We calculated hypoxia scores for 1188 tumours from 27 cancer types and showed the vast heterogeneity that exists in this microenvironmental feature within and across cancer types. This reinforces previous pushes for careful patient selection in prospective trials of hypoxia-targeting agents [16] . For the first time, we characterized the pan-cancer whole-genome correlates of tumour hypoxia. We show the broad influence of the hypoxia-associated mutator phenotype: elevated hypoxia is associated with increased mutational load across all mutational classes (i.e. CNAs, SVs and SNVs). This supports previous in vitro work that demonstrated the contextual synthetic lethality of PARP inhibition in cells with defective DNA repair due to hypoxia [39] . Regarding this co-occurrence of genomic instability and hypoxia, our group [16] and others [40] have previously described this metabolic reprogramming as a series of distinct genomic alterations. This is supported by our finding that alterations in TP53 , MYC and PTEN are more common in tumours with elevated hypoxia across cancers. Supporting these findings, previous in vitro work has shown that heterogeneous populations of cells where a small subpopulation have mutant TP53 can rapidly expand under cycling hypoxia to become the major subpopulation due to deficient apoptosis and selection [17] . We have also previously shown that tumours with TP53 mutations have elevated hypoxia within individual breast cancer subtypes, confirming that this association is not simply reflecting previously described molecular subtypes [16] . Our study cannot conclusively say whether hypoxia exerts a selective pressure that enriches for specific genomic alterations or if these genomic changes directly result in hypoxia. Experimental studies of single genes support that both effects may contribute to the associations we describe [17] , [22] , [41] , [42] , [43] . While we have not specifically included in vitro experimental validation data in this report, we and others have previously validated associations first revealed by analysis of mRNA-based hypoxia signatures. For example, our group previously described microRNA-133a-3p as a hypoxia-associated miRNA in prostate cancer based on mRNA signature-based associations across multiple independent datasets [16] . We went on to validate that microRNA-133a-3p was indeed induced under hypoxia in multiple prostate cancer cell lines and confirmed its capacity to modulate cell proliferation and invasion. Similarly, Ye et al. applied hypoxia signatures to 10 independent datasets of cell lines and primary tumour fragments under hypoxia and normoxia [44] . These 10 datasets represented seven cancer types and within each dataset samples under hypoxia showed higher hypoxia scores compared to normoxic samples. Further, they generated predictions of drugs that would be more or less potent under hypoxia and validated four drug–hypoxia interactions in vitro. These data illustrate that hypoxia signatures applied to large cohorts of primary tumours can generate reliable hypotheses, many of which have been validated in controlled systems. However, some aerobic cancer cells may also mimic the biological state of hypoxia (i.e., pseudohypoxia) and this may affect signature-derived hypoxia estimates. Further, while pimonidazole (which was used to develop the Ragnum hypoxia signature [32] ) reflects oxygen tensions below 10 mmHg (1.3% O 2 ), it is difficult to directly relate hypoxia signature scores with oxygen tension [45] . Overall, hypoxia signalling can be distinct from microenvironmental hypoxia and this remains a critical caveat of this study. Diving into the mutational processes related to hypoxia, we confirmed that several SBS and small indel signatures related to impaired DNA repair were associated with hypoxia. This raises the potential confounder that because hypoxic tumours have more mutations, we have more power to detect related mutational signatures. However, we demonstrated that hypoxia is indeed strongly associated with many mutational signatures with unknown aetiology, particularly SBS5, which is found in nearly all cancer types. Modelling these associations in vitro is particularly difficult and these data provide a high confidence measure of the mutational signatures that may be directly or indirectly driven by tumour oxygen levels. It is difficult to disentangle the timing of these events: whether a specific driver mutation gives rise to a specific mutational signature or if these are separate processes. Better mapping of the evolutionary timing of hypoxia will be particularly important in addressing this question and the advent of hypoxia signatures may facilitate future studies in this area. We observed a significant association between elevated hypoxia and the number of clonal mutations. This supports the idea that hypoxia is an early event in cancer, as we have suggested previously [16] , and other models that link hypoxia to genomic instability and downstream clonal selection [20] , [42] . Previous work has also demonstrated that patients with allelic loss of PTEN and elevated hypoxia rapidly relapse after definitive treatment for localized prostate cancer [16] . Here, we showed that tumours with alterations in PTEN and elevated hypoxia are enriched for a polyclonal tumour architecture. This illustrates the joint influence of the tumour mutational landscape and microenvironment in guiding evolutionary trajectories across cancers. Further, these data suggest that increased subclonal diversification may be a novel route via which PTEN drives aggressive tumour phenotypes, in concert with tumour hypoxia, and this can be better defined with future back-translational in vitro experiments. The PCAWG dataset is the largest publicly available pan-cancer dataset to date and this limits our ability to validate our discoveries in independent datasets. Ultimately, it will be necessary to validate our findings in large, independent cohorts. Hypotheses generated here, particularly those around hypoxia and tumour evolution, will require long term, systematic in vitro modelling and will be the subject of future studies. Overall, this work shows that a hypoxic tumour microenvironment is associated with specific mutational processes and distinct somatic mutational profiles, and may direct the subclonal architecture of cancers. Pan-cancer hypoxia scoring Hypoxia scores were calculated for all 1188 tumours with mRNA abundance data (FPKM with upper-quartile normalization) using mRNA-abundance-based signatures of tumour hypoxia developed previously by Winter et al. [31] , Buffa et al. [30] and Ragnum et al. [32] , as described previously [14] , [16] (Supplementary Data 1 ). Briefly, patients with the top 50% of mRNA abundance values for each gene in a signature were given a score of +1. Patients with the bottom 50% of mRNA abundance values for that gene were given a score of −1. This was repeated for every gene in the signature to generate a hypoxia score for each patient, and this process was repeated for each of the three signatures used in the study. High scores suggest that the tumour was hypoxic and low scores are indicative of normoxia. Hypoxia score comparison To compare hypoxia scores generated by the different signatures, the median hypoxia score was calculated for each of the PCAWG cancer types based on each signature. The median hypoxia scores from each signature were then scaled from +1 to −1 using the plotrix package (v3.7). Scaled median hypoxia values for the PCAWG cancer types were also compared to scaled median hypoxia values from previously published [16] TCGA data between comparable cancer groups. The groups compared are as follows (PCAWG cancer type and TCGA cancer type): Bladder-TCC and BLCA; Breast-AdenoCA and BRCA; Cervix-SCC and CESC; CNS-GBM and GBM; ColoRect-AdenoCA and COADREAD; Head-SCC and HNSC; Kidney-RCC and KIRC; Liver-HCC and LIHC; Lung-AdenoCA and LUAD; Lung-SCC and LUSC; Ovary-AdenoCA and OV; Panc-AdenoCA and PAAD; Prost-AdenoCA and PRAD; Skin-Melanoma and SKCM; Thy-AdenoCA and THCA; Uterus-Adeno and UCEC. Of the 27 cancer types in PCAWG, 11 (Cervix-AdenoCA, Stomach-AdenoCA, Eso-AdenoCA, Breast-LobularCA, SoftTissue-Leiomyo, Lymph-BNHL, SoftTissue-Liposarc, Biliary-AdenoCA, Kidney-ChRCC, CNS-Oligo and Lymph-CLL) did not have hypoxia data from comparable cancers in TCGA and were not used for the comparison [16] . For Spearman’s correlations, p -values were calculated using algorithm AS89. Tumour vs. normal hypoxia comparison Previously calculated pan-cancer tumour hypoxia scores were gathered for 7791 independent tumours from 19 cancer types based on the Buffa hypoxia signature [16] . Hypoxia scores were then calculated for all normal tissue samples related to the 19 cancer types with hypoxia scores ( n = 640 independent normal tissue samples). Tumour hypoxia scores were compared to normal tissue hypoxia scores for each tissue type where at least 15 normal tissue samples were available (Mann–Whitney U -test). A total of 5649 independent tumours and 625 independent normal tissue samples were evaluated in the comparisons. Linear mixed-effect models We used linear mixed-effect models to associate hypoxia with features of interest (e.g., PGA, TP53 mutational status, etc.) across cancers using the lme4 package (v1.1-17). For each feature of interest, we compared a full model (i.e., a model with the feature of interest) to a null model (i.e. a model without the feature of interest) using an ANOVA to determine if hypoxia was significantly associated with the feature of interest across cancers. A generic example of this is shown below with Eqs. ( 1 ) and ( 2 ): 
    full = hypoxia∼feature + purity + age + sex + ( 1| cancer.) (1) 
    null = hypoxia∼purity + age + sex + ( 1|cancer)
 (2) All models were adjusted for tumour purity, patient age and sex [27] , [28] . Cancer type was incorporated as a random effect in every model. This allowed us to consider a different baseline value for the feature of interest for each cancer type. For each model a conditional R 2 value is reported ( \(R_{{{\mathrm{{{LMEM - C}}}}}}^2\) ) which reflects the variance explained by the fixed and random factors [29] . We also report marginal R 2 values for each model ( \(R_{{{\mathrm{{{LMEM - M}}}}}}^2\) ) which reflect the variance explained by the fixed factors only [29] . \(R_{{{\mathrm{{{LMEM - C}}}}}}^2\) and \(R_{{{\mathrm{{{LMEM - M}}}}}}^2\) values were calculated as described previously [29] . All model diagnostics were done using the DHARMa package (0.2.0) which uses a simulation-based approach to create standardized residuals [46] . For each model, scaled residuals were generated using the simulateResiduals function. The full model was used as the input for fittedModel parameter and 1000 simulations were run. For correctly specified models, the scaled residuals were expected to be uniformly distributed and this was verified for each full model. We also compared the standardized residuals to the rank transformed predicted values to assess deviations from uniformity for each full model. Mutational density analysis Previously published data for 15 mutational density and summary features were downloaded for 1188 tumours [33] . We used linear mixed-effect models to associate each feature with hypoxia score across cancers and compared each full model with a null model. Cancer type was incorporated as a random effect in each model while tumour purity, age and sex were incorporated as fixed effects. Tumours belonging to cancer types with fewer than 15 samples were excluded from the analysis. A Bonferroni p -value adjustment was applied to the p -values from linear mixed-effect modelling since fewer than 20 tests were conducted. All models were adjusted for tumour purity based on previously published purity data [33] . The full model for evaluating PGA is shown below as an example as follows: 
    full_PGA = hypoxia∼PGA + purity + age + sex + ( 1|cancer)
 (3) To assess if SNVs per megabase were independently associated with hypoxia after adjusting for the total number of deletions we created two linear mixed-effect models. The full model associated hypoxia with SNVs per megabase while adjusting for cancer type, age, sex, tumour purity and the number of deletions (Eq. ( 4 )). For comparison, a null model was created without our feature of interest, SNVs per megabase (Eq. ( 5 )). The two models were compared using an ANOVA. [ full = hypoxia∼SNVs per megabase + purity + age + sex;                      +  total deletions + ( 1|cancer) ]
 (4) 
    null = hypoxia∼purity + age + sex +total deletions + ( 1|cancer)
 (5) Driver mutations analysis Data for driver mutations was first summarized at the gene level for 1096 tumours with previously published driver mutation data [25] . For each of the 653 driver features, we summarized if a patient had an SNV, CNA or SV. Some tumours had more than one type of event in a gene (e.g. a CNA and an SNV) and these events were classified as compound events. We then used linear mixed-effect models to associate the mutational status of each gene with hypoxia score and compared each full model with a null model. Cancer type was incorporated as a random effect in each model while tumour purity, age and sex were incorporated as fixed effects. The driver mutation analysis did not specifically consider the type of mutation in the gene and only considered if the gene had a mutation or was wildtype. Tumours belonging to cancer types with fewer than 15 samples were excluded from the analysis. An FDR adjustment was applied to the p -values from linear mixed-effect modelling. The full model for evaluating PTEN is shown below as an example as follows: 
    full_PTEN = hypoxia∼PTEN + purity + age + sex + ( 1|cancer)
 (6) Mutational signature analysis Previously published data for mutations attributed to various specific signatures was downloaded for 1188 tumours [35] . For each tumour, we calculated the proportion of total mutations attributed to each mutational signature. The proportion of mutations attributed to each signature were calculated by dividing the number of mutations attributed to each signature by the total number of mutations in the tumour. We used linear mixed-effect models to associate the proportion of mutations attributed to each signature with hypoxia score and compared each full model with a null model. Cancer type was incorporated as a random effect in each model while purity, age and sex were incorporated as fixed effects. Tumours belonging to cancer types with fewer than 15 samples were excluded from the analysis. An FDR adjustment was applied to the p -values from linear mixed-effect modelling. The full model for SBS1 is shown below as an example as follows: 
    full_SBS1 = hypoxia∼SBS1 + purity + age + sex + ( 1|cancer)
 (7) Subclonality analysis Previously reported [38] subclonal reconstruction data was used to summarize the number of clonal and subclonal mutations in all 1188 tumours. We used linear mixed-effect models to associate the number of these timed mutations with hypoxia score and compared each full model with a null model. Cancer type was incorporated as a random effect in each model while purity, age and sex were incorporated as fixed effects. Tumours belonging to cancer types with fewer than 15 samples were excluded from the analysis. A Bonferroni adjustment was applied to the p -values from linear mixed-effect modelling since fewer than 20 tests were conducted. The number of subclones was calculated for all 1188 tumours based on the number of clusters of cells identified in each sample. A linear mixed-effects model was used to associate the number of subclones with hypoxia score and this model was compared to a null model. Cancer type was incorporated as a random effect while purity, age and sex were incorporated as fixed effects. Tumours belonging to cancer types with fewer than 15 samples were excluded from the analysis. The full model for associating the number of subclones with hypoxia score is shown below as follows: 
    full_subclones = hypoxia∼subclones + purity + age + sex + ( 1|cancer)
 (8) Patients with only one identified cluster of cells were defined as monoclonal and patients with more than one identified cluster of cells were defined as polyclonal [37] . Hypoxia scores were median dichotomized to classify patients as hypoxic or normoxic. To test for an interaction between tumour hypoxia and PTEN mutational status in selecting for a particular subclonal architecture, we used linear mixed-effect models together with an ANOVA. An interaction model was first created where the relationship between the hypoxia scores and PTEN mutational status was modelled as an interaction (Eq. ( 9 )). An additive model was also created where the relationship between hypoxia scores and PTEN mutational status was modelled in an additive manner (Eq. ( 10 )): 
    interaction = clonality∼hypoxia∗PTEN + purity + age + sex + ( 1|cancer)
 (9) 
    additive = clonality∼hypoxia + PTEN + purity + age + sex + ( 1|cancer)
 (10) The two models were compared using an ANOVA to test if hypoxia scores significantly interact with PTEN mutational status. Tumours belonging to cancer types with fewer than 15 samples were excluded from the analysis. The full model diagnostics were carried out using the DHARMa package, as described above. All data analysis was performed in the R statistical environment (v3.4.3). Data visualization was performed using the BPG package [47] (v5.9.1). Figures were compiled using Inkscape (v0.91). Reporting summary Further information on research design is available in the Nature Research Reporting Summary linked to this article.